Quantum correlations with no causal order The idea that events obey a definite causal order is deeply rooted in our understanding of the world and at the basis of the very notion of time. But where does causal order come from, and is it a necessary property of nature? Here, we address these questions from the standpoint of quantum mechanics in a new framework for multipartite correlations that does not assume a pre-defined global causal structure but only the validity of quantum mechanics locally. All known situations that respect causal order, including space-like and time-like separated experiments, are captured by this framework in a unified way. Surprisingly, we find correlations that cannot be understood in terms of definite causal order. These correlations violate a 'causal inequality' that is satisfied by all space-like and time-like correlations. We further show that in a classical limit causal order always arises, which suggests that space-time may emerge from a more fundamental structure in a quantum-to-classical transition. One of the striking features of quantum mechanics is that it challenges the view that physical properties are well defined before and independent of their measurement. This motivates an operational approach to the theory, where primitive laboratory procedures, such as measurements and preparations, are basic ingredients. Although significant progress has recently been made in this direction [1] , [2] , [3] , [4] , [5] , [6] , [7] , [8] , most approaches still retain a notion of space-time as a pre-existing 'stage' in which events take place. Even the most abstract constructions, in which no explicit reference to space-time is made, do assume a definite order of events: if a signal is sent from an event A to an event B in the run of an experiment, no signal can be sent in the opposite direction in that same run. But are space, time and causal order truly fundamental ingredients of nature? Is it possible that, in some circumstances, even causal relations would be 'uncertain', similarly to the way other physical properties of quantum systems are [9] ? Here, we show that quantum mechanics allows for such a possibility. We develop a framework that describes all correlations that can be observed by two experimenters under the assumption that in their local laboratories physics is described by the standard quantum formalism, but without assuming that the laboratories are embedded in any definite causal structure. These include non-signalling correlations arising from measurements on a bipartite state, as well as signalling ones, which can arise when a system is sent from one laboratory to another through a quantum channel. We find that, surprisingly, more general correlations are possible, which are not included in the standard quantum formalism. These correlations are incompatible with any underlying causal structure: they allow performing a task—the violation of a 'causal inequality'—that is impossible if events take place in a causal sequence. This is directly analogous to the famous violation of local realism: quantum systems allow performing a task—the violation of Bell's inequality [10] —that is impossible if the measured quantities have pre-defined local values. The inequality considered here, unlike Bell's, concerns signalling correlations: it is based on a task that involves communication between two parties. Nevertheless, it cannot be violated if this communication takes place in a causal space-time. Previous works about relativistic causality in quantum mechanics focused on non-signalling correlations between space-like separated experiments or on a finite speed of signalling [11] , [12] , [13] , [14] , [15] , [16] , [17] , [18] , [19] . In the present work, we go beyond such approaches as we do not assume the existence of a space-time (or more generally of a definite causal structure) on which the evolution of quantum systems and the constraints given by relativity are defined. One of the motivations for our approach comes from the problem of time in attempts to merge quantum theory and general relativity into a more fundamental theory [20] , [21] , [22] , [23] , [24] , [25] . Causal inequality The general setting that we consider involves a number of experimenters—Alice, Bob and others—who reside in separate laboratories. At a given run of the experiment, each of them receives a physical system (for instance, a spin-1/2 particle) and performs operations on it (for example, measurements or rotations of the spin), after which she/he sends the system out of the laboratory. We assume that during the operations of each experimenter, the respective laboratory is isolated from the rest of the world—it is only opened for the system to come in and to go out, but between these two events it is kept closed. It is easy to see that, under this assumption, causal order puts a restriction on the way in which the parties can communicate during a given run. For instance, imagine that Alice can send a signal to Bob. (Formally, sending a signal (or signalling) is the existence of statistical correlations between a random variable that can be chosen by the sender and another one observed by the receiver.) As Bob can only receive a signal through the system entering his laboratory, this means that Alice must act on her system before that. But this implies that Bob cannot send a signal to Alice as each party receives a system only once. Therefore, bidirectional signalling is forbidden. Consider, in particular, the following communication task to be performed by two parties, Alice and Bob. After a given party receives the system in her/his laboratory, she/he will have to toss a coin (or use any other means) to obtain a random bit. Denote the bits generated by Alice and Bob in this way by a and b , respectively. In addition, Bob will have to generate another random bit b ′ , whose value, 0 or 1, will specify their goal: if b ′ =0, Bob will have to communicate the bit b to Alice, whereas if b ′ =1, he will have to guess the bit a . Without loss of generality, we will assume that the parties always produce a guess, denoted by x and y for Alice and Bob, respectively, for the bit of the other (although the guess may not count depending on the value of b ′ ). Their goal is to maximize the probability of success If all events obey causal order, no strategy can allow Alice and Bob to exceed the bound Indeed, as argued above, in any particular order of events, there can be at most unidirectional signalling between the parties, which means that at least one of the following must be true: Alice cannot signal to Bob or Bob cannot signal to Alice. Consider, for example, a case where Bob cannot signal to Alice. Then, if b − =1, they could in principle achieve up to P ( y = a | b′ − =1)=1 (for instance, if Alice operates on her system before Bob, she could encode information about the bit a in the system and send it to him). However, if b′ − =0, the best guess that Alice can make is a random one, resulting in P ( x = b | b′ − =0)=1/2 (see Fig. 1a ). Hence, the overall probability of success in this case will satisfy p succ ≤3/4. The same holds if Alice cannot signal to Bob. It is easy to see that no probabilistic strategy can increase the probability of success. 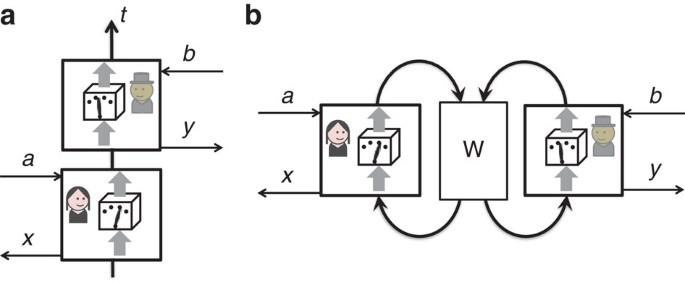Figure 1: Strategy for accomplishing communication task by using processes with definite and indefinite causal order. (a) There exists a global background time according to which Alice's actions are strictly before Bob's. She sends her inputato Bob, who can read it out at some later time and give his estimatey=a. However, Bob cannot send his bitbto Alice as the system passes through her laboratory at some earlier time. Consequently, she can only make a random guess of Bob's bit. This results in a probability of success of 3/4. (b) If the assumption of a definite order is dropped, it is possible to devise a resource (that is, a process matrixW) and a strategy that enables a probability of success(see text). Figure 1: Strategy for accomplishing communication task by using processes with definite and indefinite causal order. ( a ) There exists a global background time according to which Alice's actions are strictly before Bob's. She sends her input a to Bob, who can read it out at some later time and give his estimate y = a . However, Bob cannot send his bit b to Alice as the system passes through her laboratory at some earlier time. Consequently, she can only make a random guess of Bob's bit. This results in a probability of success of 3/4. ( b ) If the assumption of a definite order is dropped, it is possible to devise a resource (that is, a process matrix W ) and a strategy that enables a probability of success (see text). Full size image Formally, the assumptions behind the causal inequality (2) can be summarized as follows: Causal structure The main events in the task (a system entering Alice's/Bob's laboratory, the parties obtaining the bits a , b and b ′, and producing the guesses x and y ) are localized in a causal structure. A causal structure (such as space-time) is a set of event locations equipped with a partial order that defines the possible directions of signalling. If A B , we say that A is in the causal past of B (or B is in the causal future of A ). In this case, signalling from A to B is possible, but not from B to A . For more details on causal structures, see Supplementary Methods . Free choice Each of the bits a , b and b can only be correlated with events in its causal future (this concerns only events relevant to the task). We assume also that each of them takes values 0 or 1 with probability 1/2. Closed laboratories Alice's guess x can be correlated with Bob's bit b only if the latter is generated in the causal past of the system entering Alice's laboratory. Analogously, y can be correlated with a only if a is generated in the causal past of the system entering Bob's laboratory. In the Supplementary Methods , we present a formal derivation of the inequality from these assumptions.Interestingly, we find that if the local laboratories are described by quantum mechanics, but no assumption about a global causal structure is made ( Fig. 1b ), it is in principle possible to violate the causal inequality in physical situations in which one would have all the reasons to believe that the bits are chosen freely and the laboratories are closed. This would imply that the assumption Causal structure does not hold. Framework for local quantum mechanics The most studied, almost epitomical, quantum correlations are the non-signalling ones, such as those obtained when Alice and Bob perform measurements on two entangled systems. Signalling quantum correlations exist as well, such as those arising when Alice operates on a system that is subsequently sent through a quantum channel to Bob who operates on it after that. The usual quantum formalism does not consider more general possibilities, as it does assume a global causal structure. Here, we want to drop the latter assumption while retaining the validity of quantum mechanics locally. For this purpose, we consider a multipartite setting of the type outlined earlier, where each party performs an operation on a system passing once through her/his laboratory, but we make no assumption about the spatio-temporal location of these experiments, not even that there exists a space-time or any causal structure in which they could be positioned (see Fig. 2 ). Our framework is thus based on the central premise of local quantum mechanics, which is to say the local operations of each party are described by quantum mechanics. 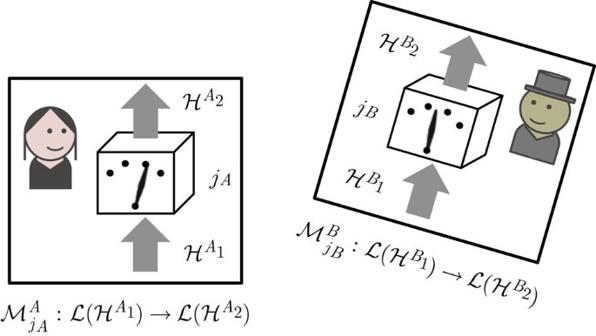Figure 2: Local quantum experiments with no assumption of a pre-existing background time or global causal structure. Although the global causal order of events in the two laboratories is not fixed in advance and in general not even definite (here illustrated by the 'shifted' relative orientation of the two laboratories), the two agents, Alice and Bob, are each certain about the causal order of events in their respective laboratories. Figure 2: Local quantum experiments with no assumption of a pre-existing background time or global causal structure. Although the global causal order of events in the two laboratories is not fixed in advance and in general not even definite (here illustrated by the 'shifted' relative orientation of the two laboratories), the two agents, Alice and Bob, are each certain about the causal order of events in their respective laboratories. Full size image More specifically, we assume that one party, say Alice, can perform all the operations she could perform in a closed laboratory, as described in the standard space-time formulation of quantum mechanics. These are defined as the set of quantum instruments [26] with an input Hilbert space (the system coming in) and an output Hilbert space (the system going out). (The set of allowed quantum operations can be used as a definition of 'closed quantum laboratory' with no reference to a global causal structure.) A quantum instrument can most generally be realized by applying a joint unitary transformation on the input system plus an ancilla, followed by a projective measurement on part of the resulting joint system, which leaves the other part as an output. (From the point of view of each party, the input/output systems most generally correspond to two subsystems of the Hilbert space associated with the local laboratory, each considered at a different instant—the time of entrance and the time of exit, respectively—where the subsystems and the respective instants are independent of the choice of operation that connects them.) When Alice uses a given instrument, she registers one out of a set of possible outcomes, labelled by j =1,..., n . Each outcome induces a specific transformation from the input to the output, which corresponds to a completely positive (CP) trace-non-increasing map [27] , where , is the space of matrices over a Hilbert space of dimension d X . The action of each on any matrix can be written as [27] , where the matrices satisfy , ∀ j . If the operation is performed on a quantum state described by a density matrix ρ, describes the updated state after the outcome j up to normalization, whereas the probability to observe this outcome is given by . The set of CP maps corresponding to all the possible outcomes of a quantum instrument has the property that is CP and trace-preserving (CPTP) or equivalently , which reflects the fact that the probability to observe any of the possible outcomes is unity. A CPTP map itself corresponds to an instrument with a single outcome that occurs with certainty. In the case of more than one party, the set of local outcomes corresponds to a set of CP maps . A complete list of probabilities for all possible local outcomes will be called process. (It is implicitly assumed that the joint probabilities are non-contextual, namely that they are independent of any variable concerning the concrete implementation of the local CP maps. For example, the probability for a pair of maps to be realized should not depend on the particular set of possible CP maps associated with Alice's operation.) A process can be seen as an extension of the notion of state as a list of probabilities for detection results [3] described by a positive operator-valued measure (POVM), which takes into account the transformation of the system after the measurement and can thus capture more general scenarios than just detection. Here, we will consider explicitly only the case of two parties (the generalization to arbitrarily many parties is straightforward). We want to characterize the most general probability distributions for a pair of outcomes i , j , corresponding to CP maps , to be observed, that is, to characterize all bipartite processes. In quantum mechanics, operations obey a specific algebraic structure that reflects the operational relations between laboratory procedures [3] . For example, a probabilistic mixture of operations is expressed as a linear convex combination of CP maps. It can be shown (see Methods) that the only probabilities consistent with the algebraic structure of local quantum operations are bilinear functions of the CP maps and . Thus, the study of the most general bipartite quantum correlations reduces to the study of bilinear functions of CP maps. It is convenient to represent CP maps by positive semi-definite matrices via the Choi-Jamiołkowsky (CJ) isomorphism [28] , [29] . The CJ matrix coresponding to a linear map is defined as , where is a (not normalized) maximally entangled state, the set of states is an orthonormal basis of is the identity map and T denotes matrix transposition (the transposition, absent in the original definition, is introduced for later convenience). Using this correspondence, the probability for two measurement outcomes can be expressed as a bilinear function of the corresponding CJ operators as follows: where is a matrix in . The matrix W should be such that probabilities are non-negative for any pair of CP maps . We require that this be true also for measurements in which the system interacts with any system in the local laboratory, including systems entangled with the other laboratory. This implies that must be positive semidefinite (see Methods). Furthermore, the probability for any pair of CPTP maps to be realized must be unity (they correspond to instruments with a single outcome). As a map is CPTP if and only if its CJ operator satisfies and (similarly for ), we conclude that all bipartite probabilities compatible with local quantum mechanics are generated by matrices W that satisfy We will refer to a matrix that satisfies these conditions as a process matrix. Conditions equivalent to equations (4) and (5) were first derived as part of the definition of a 'quantum comb' [30] , an object that formalizes quantum networks. Combs, however, are subject to additional conditions fixing a definite causal order, which are not assumed here. A process matrix can be understood as a generalization of a density matrix and equation (3) can be seen as a generalization of Born's rule. In fact, when the output systems A 2 , B 2 are taken to be one-dimensional (that is, each party performs a measurement after which the system is discarded), the expression above reduces to , where now are elements of local POVMs and is a quantum state. This implies that a quantum state shared by Alice and Bob is generally represented by the process matrix . Signalling correlations can also be expressed in terms of process matrices. For instance, the situation where Bob is given a state and his output is sent to Alice through a quantum channel , which gives , is described by , where is the CJ matrix of the channel from B 2 to A 1 . The most general bipartite situation typically encountered in quantum mechanics (that is, one that can be expressed in terms of a quantum circuit) is a quantum channel with memory, where, say, Bob operates on one part of an entangled state and his output plus the other part is transferred to Alice through a channel. This is described by a process matrix of the form . Conversely, all process matrices of this form represent channels with memory [30] . This is the most general situation in which signalling from Alice to Bob is not possible, a relation that we will denote by in accord with the causal notation introduced earlier. Process matrices of this kind will be denoted by (note that for non-signalling processes, both and are true). As argued earlier, if all events are localized in a causal structure, and Alice and Bob perform their experiments inside closed laboratories, at most unidirectional signalling between the laboratories is allowed. In a definite causal structure, it may still be the case that the location of each event, and thus the causal relation between events, is not known with certainty. A situation where with probability 0≤ q ≤1 and with probability 1− q is represented by a process matrix of the form We will call the processes of this kind causally separable (note that the decomposition (6) need not be unique as non-signalling processes can be included either in or in ). They represent the most general bipartite quantum processes for which the local experiments are performed in closed laboratories embedded in a definite causal structure. In particular, they generate the most general quantum correlations between measurements that take place at definite (though possibly unknown) instants of time. Clearly, according to the argument presented earlier, causally separable processes cannot be used by Alice an Bob to violate the causal inequality (2). In the Supplementary Methods , we provide a complete characterization of process matrices via the terms allowed in their expansion in a Hilbert–Schmidt basis, which we relate to the possible directions of signalling they allow (see Fig. 3 ). We also provide possible interpretations of the terms that are not allowed in a process matrix (see Fig. 4 and Supplementary Fig. S1 ). 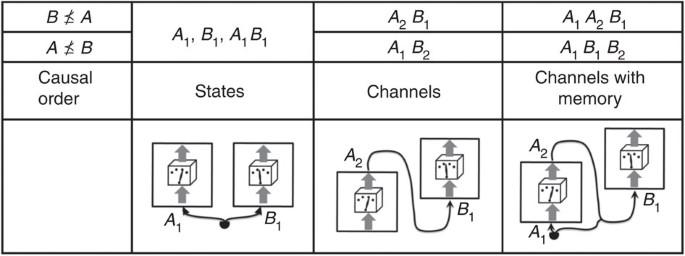Figure 3: Terms appearing in a process matrix. A matrix satisfying condition (4) can be expanded as, where the set of matrices, withandfor, provide a basis of. We refer to terms of the formas of the typeA1, terms of the formas of the typeA1A2and so on. In theSupplementary Information, we prove that a matrix satisfies condition (5) if it contains the terms listed in this table. Each of the terms can allow signalling in at most one direction and can be realized in a situation in which either Bob's actions are not in the causal past of Alice'sor vice versa. The most general unidirectional process is a quantum channel with memory. Measurements of bipartite states that lead to non-signalling probabilities can be realized in both situations. The most general process matrix can contain terms from both rows and may not be decomposable into a mixture of quantum channels from Alice to Bob and from Bob to Alice. Figure 3: Terms appearing in a process matrix. A matrix satisfying condition (4) can be expanded as , where the set of matrices , with and for , provide a basis of . We refer to terms of the form as of the type A 1 , terms of the form as of the type A 1 A 2 and so on. In the Supplementary Information , we prove that a matrix satisfies condition (5) if it contains the terms listed in this table. Each of the terms can allow signalling in at most one direction and can be realized in a situation in which either Bob's actions are not in the causal past of Alice's or vice versa . The most general unidirectional process is a quantum channel with memory. Measurements of bipartite states that lead to non-signalling probabilities can be realized in both situations. The most general process matrix can contain terms from both rows and may not be decomposable into a mixture of quantum channels from Alice to Bob and from Bob to Alice. 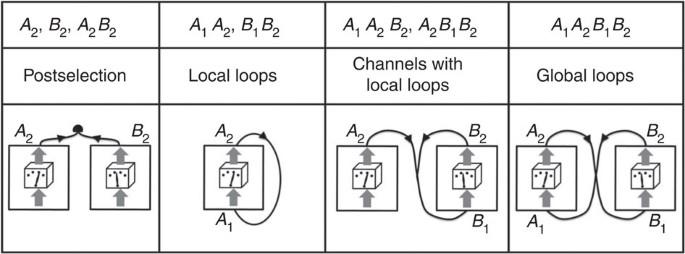Figure 4: Terms not appearing in a process matrix. These terms are not compatible with local quantum mechanics because they yield non-unit probabilities for some CPTP maps. A possible interpretation of these terms within our framework is that they correspond to statistical sub-ensembles of possible processes. For example, terms of the typeA2can be understood as postselection. One specific case is when a system enters a laboratory in a maximally mixed state, is subject to the mapMand, after going out of the laboratory, is measured to be in some state |ψ . The corresponding probability is given by, generated in our formalism by. Notably, correlations of the typeA1A2have been exploited in models for describing CTCs43,45. The pictures are only suggestive of the possible interpretations. Full size image Figure 4: Terms not appearing in a process matrix. These terms are not compatible with local quantum mechanics because they yield non-unit probabilities for some CPTP maps. A possible interpretation of these terms within our framework is that they correspond to statistical sub-ensembles of possible processes. For example, terms of the type A 2 can be understood as postselection. One specific case is when a system enters a laboratory in a maximally mixed state, is subject to the map M and, after going out of the laboratory, is measured to be in some state |ψ . The corresponding probability is given by , generated in our formalism by . Notably, correlations of the type A 1 A 2 have been exploited in models for describing CTCs [43] , [45] . The pictures are only suggestive of the possible interpretations. Full size image A causally non-separable process The question whether all local quantum experiments can be embedded in a global causal structure corresponds to the question whether all process matrices are causally separable. Note that this is not a question about entanglement: all possible entangled states, and more generally all quantum circuits, correspond to matrices of the form or , whereas the non-separable processes we are looking for cannot be written as quantum circuits or even as probabilistic mixtures of different circuits. Surprisingly, an example of such a kind exists. Consider the process matrix where A 1 , A 2 , B 1 and B 2 are two-level systems (for example, the spin degrees of freedom of a spin- particle) and σ x and σ z are the Pauli spin matrices. It can be verified straightforwardly that conditions (4) and (5) are satisfied, hence (7) is a valid bipartite process. Having such a resource, Alice and Bob can play the game described above and exceed the bound on the probability of success (2) imposed by causal order. Indeed, if Bob measures in the z basis and detects one of the states | z ± 〉, the corresponding CJ operator contains the factor . Inserting this, together with equation (7), into the expression (3) for the probabilities, the term containing in the process matrix is annihilated and what remains corresponds to a noisy channel from Alice to Bob. If Alice encodes her bit in the z basis with the CJ operator , this channel allows Bob to guess Alice's bit with probability . If, on the other hand, Bob measures in the x basis, equation (7) is reduced to a similar noisy channel from Bob to Alice. Bob is thus able to activate a channel in the desired direction by choosing the measurement basis (see Methods for a detailed calculation and analysis of the protocol). In this way they can achieve which proves that (7) is not causally separable. We see that, depending on his choice, Bob can effectively end up 'before' or 'after' Alice, each possibility with a probability . This is remarkable, because if Alice and Bob perform their experiments inside laboratories that they believe are isolated from the outside world for the duration of their operations (for example, by walls made of impenetrable material), and if they believe that they are able to freely choose the bits a , b and b ' (for example, by tossing a coin), they will have to conclude that the events in their experiment do not take place in a causal sequence. Indeed, the framework only assumes that the local operations from the input to the output system of each party are correctly described by quantum mechanics, and it is compatible with any physical situation in which one would have all the reasons to believe that each party's operations are freely chosen in a closed laboratory. Interestingly, both the classical bound (2) and the quantum violation (8) match the corresponding numbers in the CHSH-Bell inequality [31] , which strongly resembles inequality (2). However, the physical situations to which these inequalities correspond is very different: Bell inequalities can be violated in space-like separated laboratories, while (8) cannot be achieved neither with space-like nor with time-like separated laboratories. It is an open question whether (8) is the maximal possible violation allowed by quantum mechanics. Classical processes are causally separable It is not difficult to see that if the operations of the local parties are classical, they can always be understood as taking place in a global causal structure. Classical operations can be described by transition matrices , where P (λ 2 , j |λ 1 ) is the conditional probability that the measurement outcome j is observed and the classical output state λ 2 is prepared given that the input state is λ 1 . They can be expressed in the quantum formalism as CP maps diagonal in a fixed ('pointer') basis, and the corresponding CJ operators are . Thus, to express arbitrary bipartite probabilities of classical maps, it is sufficient to consider process matrices that are diagonal in the pointer basis. In the Supplementary Methods, we provide a detailed proof that all such processes are causally separable. We have seen that by relaxing the assumption of definite global causal order and requiring that the standard quantum formalism holds only locally, we obtain the possibility for global causal relations that are not included in the usual formulation of quantum mechanics. The latter is reminiscent of the situation in general relativity, where by requiring that locally the geometry is that of flat Minkowski space-time, one obtains the possibility of having more general, curved space-times. The natural question is whether 'non-causal' quantum correlations of the kind described by our formalism can be found in nature. One can speculate that they may exist in unprobed physical regimes, such as, for example, those in which quantum mechanics and general relativity become relevant. Indeed, our result that classical theories can always be understood in terms of a global causal structure suggests the possibility that the observed causal order of space-time might not be a fundamental property of nature but rather emerge from a more fundamental theory [32] , [33] , [34] in a quantum-to-classical transition due to, for example, decoherence [35] or coarse-grained measurements [36] . Once a causal structure is present, it is possible to derive relativistic space-time from it under appropriate conditions [37] , [38] . Furthermore, as the conformal space-time metric is a description of the causal relation between space-time points [39] , [40] , one can expect that an extension of general relativity to the quantum domain would involve situations where different causal orders could coexist 'in superposition'. The formalism we presented may offer a natural route in this direction: based only on the assumption that quantum mechanics is valid locally, it yields causal relations that cannot be understood as arising from a definite, underlying order. It is also worth noting that exotic causal structures already appear in the classical theory of general relativity. For example, there exist solutions to the Einstein equation containing closed time-like curves (CTCs) [41] . In this context, it should be noted that any process matrix W in our framework can be interpreted as a CPTP map from the outputs, A 2 , B 2 , of the parties, to their inputs, A 1 , B 1 . In other words, any process can be thought of as having the form of a CTC, where information is sent back in time through a noisy channel (see also Fig. 1b ). The existence of processes that do not describe definite causal order is therefore not incompatible with general relativity in principle. It is sometimes argued that CTCs should not exist as they generate logical paradoxes, such as an agent going back in time and killing his grandfather. The possible solutions that have been proposed [42] , [43] , [44] , [45] , [46] , [47] , in which quantum mechanics and CTCs might coexist, involve non-linear extensions of quantum theory that deviate from quantum mechanics already at the level of local experiments. Our framework, on the other hand, is by construction linear and in agreement with local quantum mechanics, and yet paradoxes are avoided, in accordance with the Novikov principle [48] , due to the noise in the evolution 'backward in time'. Finally, we remark that instances of indefinite causal orders may also emerge in situations closer to possible laboratory implementations. As already noted, our formalism describes more general correlations than those that can be realized with a quantum circuit, that is, as a sequence of quantum gates. Recently, a new model of quantum computation that goes beyond the causal paradigm of quantum circuits by using superpositions of the 'wires' connecting different gates was proposed [49] . This possibility may allow breaking the assumption that events are localized in a causal structure. As the instant when a system enters a device depends on how the device is wired with the rest of the computer's architecture, superpositions of wires may allow creating situations in which events are not localized in time (similarly to the way in which a quantum particle may not be localized in space). Although it is an open question whether violating the causal inequality (2) can be achieved by similar means, the present work suggests that new quantum resources for information processing might be available—beyond entanglement, quantum memories and even 'superpositions of wires'—and the formalism introduced provides a natural framework for exploring them. Definition of process matrices In this section, we will derive the linear representation (3), as well as the conditions (4) and (5) that a process matrix has to satisfy. Linearity of probabilities A quantum instrument [26] is defined as a set of CP maps such that is a CPTP map. Our main assumption is that the description of the operations in the individual laboratories is in agreement with quantum mechanics. In particular, we derive linearity from the quantum mechanical representation of probabilistic mixtures and of coarse-graining of operations. Consider first an instrument defined as the randomization of two different instruments and , where the first is performed with probability p and the second with probability (1− p ). The probability to observe the outcome j is, by definition, . In quantum mechanics, randomization is described as a convex linear combination, . We can then conclude that the probability must respect linear convex combinations: . Consider then the coarse-graining of an instrument . This is realized when two or more outcomes, for example, those corresponding to the labels j = n −1 and j = n , are treated as a single one. In the resulting instrument , all non-coarse-grained outcomes correspond to the original CP maps , whereas the probability of the coarse-grained outcome is given by . In quantum mechanics, the CP map corresponding to the coarse graining of two outcomes is represented by the sum of the respective CP maps, , from which it follows that . Randomization and coarse graining together impose linearity. The argument can be repeated for two (or more) parties, yielding the conclusion that all bipartite probabilities compatible with a local quantum mechanical description are bilinear functions, , of the local CP and trace-non-increasing maps . Thanks to the CJ isomorphism, it is possible to represent bilinear functions of CP maps as bilinear functions of matrices: . In general, multilinear functions on a set of vector spaces V 1 × V 2 ×... are isomorphic to linear functions on , hence the probabilities can be written as linear functions on . Using the Hilbert–Schmidt scalar product, we can identify each real linear function with an element of the same space, , arriving at the representation (3). Non-negativity and normalization of probabilities The requirement that the probabilities are non-negative for any pair of CP maps and imposes the restriction that W is positive on pure tensors [50] with respect to the partition A 1 A 2 − B 1 B 2 . These are matrices such that The condition has to be imposed for arbitrary positive semidefinite matrices and because these are the CJ matrices of CP maps. We additionally assume that the parties can share arbitrary (possibly entangled) ancillary states independent of the process, and use them in their local operations. The latter means that each party can extend the input space of her/his operations to the ancillas, which we denote by and for Alice and Bob, respectively, and apply arbitrary quantum operations with CP maps . (One can similarly extend the output systems, but this is not necessary for our argument.) The assumption that the ancillary systems contain a joint quantum state independent of the process means that if separate operations are applied on the ancillas and the original systems, the joint probability distribution for the outcomes is a product of two distributions—one for the outcomes on the ancillas, which is the same as one arising from a measurement on a quantum state , and another one for the outcomes on the original systems, which is given by equation (3) with the original . These requirements imply that the extended process matrix is given by . If we then require that the probabilities for extended operations are non-negative, one has It was shown [50] that condition (10) is satisfied if and only if is positive semidefinite (a class strictly smaller than positive on pure tensors), which is condition (4). Additionally, probabilities must be normalized: , which means Condition (5) can be deduced from equation (11) simply by noticing that for a CPTP map M the corresponding CJ matrix satisfies the condition . To see that this is also a sufficient condition for a map to be trace-preserving, it is enough to consider the inverse direction of the CJ isomorphism, Violation of the causal inequality The process described by equation (7) can be exploited for the task described above in the following way. Alice always measures the incoming qubit in the z basis, assigning the value x =0 to the outcome | z + 〉 and x =1 to | z − 〉. She then reprepares the qubit, encoding a in the same basis, and sends it away. It is easy to see that the CP map corresponding to the detection of a state |ψ〉 and repreparation of another state |φ〉 has CJ matrix . Accordingly, the possible operations performed by Alice can be represented compactly by the CJ matrix Bob adopts the following protocol. If he wants to read Alice's bit ( b ′ =1), he measures the incoming qubit in the z basis and assigns y =0, y =1 to the outcomes | z + 〉, | z − 〉, respectively (the repreparation is unimportant in this case). If he wants to send his bit ( b ′=0), he measures in the x basis, and if the outcome is | x + 〉, he encodes b in the z basis of the outgoing qubit as 0→| z + 〉, 1→| z − 〉, whereas if the outcome is | x − 〉, he encodes it as 0→| z − 〉, 1→| z + 〉. The CJ matrix representing Bob's CP map is where is the arbitrary state prepared when b ′=1 (with ) and ⊕ denotes the sum modulo 2. Note that in equation (16), Bob's assignment | x + 〉→ y =0, | x − 〉→ y =1 for the outcome of his measurement is arbitrary, because for b ′=0 he is not trying to correlate y with a . The probabilities for different possible outcomes, when the described protocol is applied to the process (7), are given, according to (3), by . To calculate the success probability, we need as intermediate steps and . Notice that when the outcome of one party is ignored, it is always possible to identify a specific state in which the other party receives the qubit. For example, to average out Alice's outcomes one has to calculate The process observed by Bob is therefore described by the reduced matrix The matrix represents the CPTP map performed by Alice when the outcomes of her measurement are ignored (the explicit dependence on a accounts for the possibility of signalling). Using (13), we find , which, plugged into equation (17) together with equation (7), gives When this is measured with the map (15), we find from which we obtain . Consider now the case when b ′ =0. When Bob's outcomes are ignored, he performs the CPTP map described by . From this we can calculate, as in the previous case, the effective state received by Alice, which is from which we find . In conclusion, the protocol described yields the probability of success (8), which proves that the process in equation (7) is not causally separable. How to cite this article: Oreshkov, O. et al . Quantum correlations with no causal order. Nat. Commun. 3:1092 doi: 10.1038/ncomms2076 (2012).